An elasto-mechanical unfeelability cloak made of pentamode metamaterials Metamaterial-based cloaks make objects different from their surrounding appear just like their surrounding. To date, cloaking has been demonstrated experimentally in many fields of research, including electrodynamics at microwave frequencies, optics, static electric conduction, acoustics, fluid dynamics, thermodynamics and quasi two-dimensional solid mechanics. However, cloaking in the seemingly simple case of three-dimensional solid mechanics is more demanding. Here, inspired by invisible core-shell nanoparticles in optics, we design an approximate elasto-mechanical core-shell ‘unfeelability’ cloak based on pentamode metamaterials. The resulting three-dimensional polymer microstructures with macroscopic overall volume are fabricated by rapid dip-in direct laser writing optical lithography. We quasi-statically deform cloak and control samples in the linear regime and map the displacement fields by autocorrelation-based analysis of recorded movies. The measured and the calculated displacement fields show very good cloaking performance. This means that one can elastically hide objects along these lines. Artificial materials called metamaterials [1] , [2] or composites [3] have significantly improved our ability to steer waves and energy fluxes in electromagnetism, optics, acoustics, thermodynamics and mechanics. Invisibility cloaks [4] , [5] , [6] , [7] and counterparts thereof are demonstrations of this progress. Cloaks have been demonstrated experimentally in electromagnetism at microwave [8] and at optical frequencies [9] , [10] , [11] , in airborne [12] , [13] and fluid-borne acoustics [14] , for fluid surface waves [15] , for electrical [16] and heat conduction [17] , [18] , [19] , as well as for flexural waves [20] in thin (quasi two-dimensional) elastic membranes. In three-dimensional (3D) solid mechanics, only unidirectional cloaking of stress waves in fibrous materials has been achieved [21] . What makes cloaking in 3D solid mechanics harder than cloaking in other systems? An isotropic dielectric optical material can be described by a simple scalar electric permittivity, an isotropic magnetic material by a scalar magnetic permeability, an isotropic electric (or thermal) conductor by a scalar electric (or heat) conductivity, an isotropic diffusive medium by a scalar diffusivity and so on. In contrast, in mechanics, regular 3D elastic solids can only be treated by a rank-4 elasticity tensor [22] . Even for isotropic media, it contains two independent elements, namely the material’s bulk modulus B and shear modulus G . Intuitively, these moduli describe the forces needed to change the volume and the shape of a linearly elastic material, respectively, while fixing the other. Mechanics becomes much simpler for the acoustics of gases/fluids [2] , [3] , which are defined by strictly zero shear modulus, that is, G =0. The theory underlying cloaking has either been based on analytical coordinate transformations [3] , [4] , [5] , [6] or on numerical topology optimization [13] , [23] , [24] , [25] . The analytical theory for mere invisibility and analogues thereof based on simple spherical or cylindrical core-shell geometries has been worked out a long time ago [26] , [27] , [28] . We use the core-shell approach below. Whatever the approach, a cloak—as opposed to just a ‘neutral inclusion’ that is not necessarily a cloak—makes an arbitrary object within the cloak appear just like a given surrounding. To accomplish this goal, the object needs to be isolated from the surrounding for all conditions. In optics, isolation can be achieved by an opaque metal wall, in electrical conduction by an electrically insulating wall and in heat conduction by a thermally insulating wall. In mechanics, one needs a rigid (that is, immovable) wall. Next, a suitable structure is wrapped around these walls to make them and their interior appear identical to the surrounding. A similar core-shell approach has just recently been successfully used in thermal cloaking [18] , [19] . In this paper, we experimentally demonstrate an approximate core-shell elasto-mechanical cloak. Elasto-mechanical cloak design What function does such an ‘unfeelability cloak’ serve? For example, lying on an elastic bed mattress, you would normally feel a stiff object underneath the mattress (also see illustration Supplementary Fig. 1 ). In contrast, a cloaking mattress on top of the same stiff object would appear to the outside as a homogeneous isotropic elastic solid. In this fashion, one can elastically hide objects. Inspired by invisible core-shell geometries in optics [29] , we use the mechanical core-shell approach illustrated in Fig. 1 . Theory for elastic core-shell geometries was published by Kerner [26] and later by Hashin and Shtrikman [28] . The textbook of Milton [3] comprehensively reviews the theoretical work published since then, much of which uses the notion of ‘neutral inclusions’. More recently, a theoretical optimization study has been published [30] . In Fig. 1 , we aim at statically cloaking an arbitrary object located inside a rigid (that is, ideally incompressible and not deformable) hollow cylinder with inner radius R i , outer radius R 1 , bulk modulus B 1 →∞ and shear modulus G 1 →∞. As pointed out above, this rigid wall already isolates and protects any object inside with respect to the outside. By additionally wrapping around the cylinder a homogeneous isotropic shell (with outer radius R 2 , bulk modulus B 2 and shear modulus G 2 ), we wish to make this core-shell geometry appear elastically as its isotropic compliant homogeneous surrounding (with bulk modulus B 0 and shear modulus G 0 ). 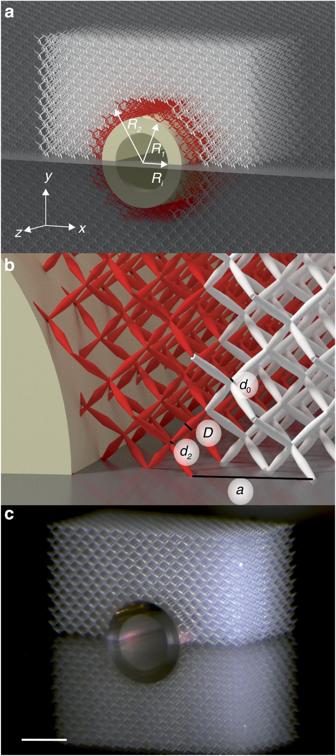Figure 1: Illustration of the elasto-mechanical cloak. (a) A rigid hollow cylinder embedded in a homogeneous three-dimensional pentamode-metamaterial environment (white) is covered by a compliant pentamode-metamaterial shell (red). Any object can be placed inside of the hollow interior and thereby becomes ‘unfeelable’. For any given pushing direction, the cylindrical core-shell geometry exhibits a symmetry plane normal to the pushing direction and cutting through the middle of the cylinder. Thus, it is sufficient to study the half-cylinder geometry. (b) The magnified view reveals the details of the pentamode metamaterial the cloak is composed of. The local bulk modulusBis tuned via the diameterdof the double-cone connections with respect to the fixed lattice constanta. For the surrounding, we chosed0/a=5.3% (white), for the cloaking shell we derived2/a=2.4% (red) for the choiceR2/R1=4/3. The fixed diameterD/a=8% at the thick ends is also depicted. (c) Optical micrograph of a fabricated cloaking structure. Scale bar, 0.5 mm. Figure 1: Illustration of the elasto-mechanical cloak. ( a ) A rigid hollow cylinder embedded in a homogeneous three-dimensional pentamode-metamaterial environment (white) is covered by a compliant pentamode-metamaterial shell (red). Any object can be placed inside of the hollow interior and thereby becomes ‘unfeelable’. For any given pushing direction, the cylindrical core-shell geometry exhibits a symmetry plane normal to the pushing direction and cutting through the middle of the cylinder. Thus, it is sufficient to study the half-cylinder geometry. ( b ) The magnified view reveals the details of the pentamode metamaterial the cloak is composed of. The local bulk modulus B is tuned via the diameter d of the double-cone connections with respect to the fixed lattice constant a . For the surrounding, we chose d 0 / a =5.3% (white), for the cloaking shell we derive d 2 / a =2.4% (red) for the choice R 2 / R 1 =4/3. The fixed diameter D / a =8% at the thick ends is also depicted. ( c ) Optical micrograph of a fabricated cloaking structure. Scale bar, 0.5 mm. Full size image To accomplish this goal, we need to make the core-shell appear as the surrounding with respect to compression as well as with respect to shear. It is the combination of these two aspects—compression and shear—that makes cloaking in mechanics harder than cloaking in other areas of physics. In regard to shear, Hashin and Shtrikman [28] showed that this necessarily requires G 1 = G 0 , from which the condition G 2 = G 1 = G 0 follows [28] . Mathematically, this condition is immediately fulfilled by any three liquids with zero shear moduli. The liquids would, however, rapidly intermix and flow away. Hence, the cloak would not be stable. A rigid isolating wall (with B 1 →∞ and G 1 →∞) requires a solid. This immediately leads to a surrounding with G 0 →∞, which is not deformable as well, and would hence not represent an impressive demonstration of cloaking at all. We conclude that the mechanical core-shell approach does not allow for perfect elasto-mechanical cloaking using a rigid wall for isolation and a compliant solid as surrounding. Nevertheless, cloaking [24] , [31] may still be possible upon simply ignoring the condition G 2 = G 1 = G 0 , in which case cloaking is no longer expected to be strict. Our approximate approach is to search for solutions based on a rigid wall, whereas the surrounding as well as the shell exhibit relatively small shear moduli. In 1995, corresponding pentamode metamaterials have independently been suggested by Sigmund [32] and by Milton and Cherkaev [33] . Bendsøe and Sigmund [32] used numerical topology optimization [25] ; Milton and Cherkaev’s [33] considerations were analytical and included anisotropic versions. Pentamode materials have a pseudo-elasticity tensor with one non-zero eigenvalue that is of the pure pressure type. Polymeric realizations of pentamode metamaterials with ratios of bulk to shear modulus as large as B / G =1,000 have recently become available experimentally in microscopic [34] and macroscopic [35] form. The pentamode microstructure [33] , [34] is illustrated in Fig. 1 . In regard to static compression, assuming an incompressible and not deformable hollow cylinder (that is, B 1 / B 0 ≫ 1, B 1 / B 2 ≫ 1, G 1 / G 0 ≫ 1 and G 1 / G 2 ≫ 1) as well as pentamode metamaterials for the surrounding (that is, B 0 / G 0 ≫ 1) and for the shell (that is, B 2 / G 2 ≫ 1), one gets the simple result [3] for the relative bulk modulus of the shell (upon using in the nomenclature of ref. 3 ) Numerical continuum-mechanics calculations (not depicted) indicate that this formula remains valid as long as the B 2 / G 2 ratio is larger than some 100. For example, choosing a thin shell with R 2 / R 1 =4/3, the formula leads to a relative bulk modulus of the shell of B 2 / B 0 =7/16≈0.44. Intuitively, the operation with respect to compression can easily be understood by analogy to a one-dimensional periodic chain of identical Hooke springs, each with finite spring constant D 0 . One spring shall now be replaced by a very stiff one, that is, D 1 →∞. To compensate for that, the two neighbouring springs with spring constant D 2 must be made softer. To become undetectable with respect to compression, the effective spring constant of the three springs must be identical to three identical springs (each with spring constant D 0 ) in series. One immediately gets D 2 / D 0 =2/3. In three dimensions, however, the situation is more complex because a compression of an elastic solid in one direction is accompanied by an expansion/contraction in the two orthogonal directions. This makes the problem non-trivial. Next, we map these parameters onto a pentamode microstructure (see Fig. 1 ). The bulk modulus can be tailored via the ratio of the small connection diameter d and the face-centered cubic (fcc) unit cell lattice constant a (see Fig. 1 ). For simplicity, we also fix the diameter D of the thick ends of the double cones throughout the entire structure as this quantity hardly enters into the mechanical properties [34] . We have previously shown [35] that the effective pentamode bulk (shear) modulus scales approximately according to B ∝ d / a and G ∝ ( d / a ) 3 . We choose a cylinder rather than a sphere because this geometry allows us to observe the displacement close to the surface of the cloaking shell as directly as possible at the samples’ boundaries. For any specific pushing direction in Fig. 1 , e.g., along the vertical direction, by symmetry, the problem is equivalent to a half of it. This geometry somewhat resembles the 3D carpet cloak demonstrated experimentally in optics a few years ago [11] . For simplicity, we use this carpet or mattress geometry (see Supplementary Fig. 1 ) in our experiments as it is clear by symmetry that the complete free-space structure is omnidirectional. Experimental results Altogether, our fabricated pentamode cloak microstructure depicted in Fig. 2 has the following design parameters: a =125 μm and D / a =8% (or D =10 μm) throughout, R i / a =2 (not critical because the wall is rigid), R 1 / a =3, R 2 / a =4, d 0 / a =5.3% (or d 0 =6.6 μm) and d 2 / a =2.4% (or d 2 =3.0 μm). Within the surrounding, this leads to B 0 / G 0 =120, in the cloaking shell to B 2 / G 2 =908. The overall polymer microstructure shown in Fig. 2 contains 16 × 8 × 8=1,024 extended fcc pentamode unit cells and has a total volume of V =2 mm 3 . Within measurement accuracy, the structure parameters a , D and d 0 are identical to their design values. Owing to fabrication constraints, only the diameter d 2 in Fig. 2f is slightly larger than its design value. The fabrication of each sample by fast galvo-scanner dip-in 3D direct laser writing (DLW) optical lithography has taken about 12 h (for details see Methods). We are not aware of any other approach capable of yielding structures with such small internal and such large overall dimensions. 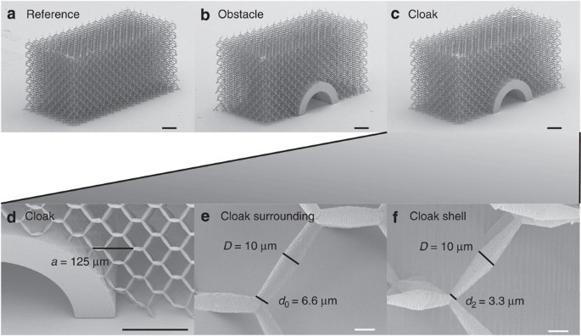Figure 2: Fabricated elasto-mechanical structures. Electron micrographs of (a) the homogeneous pentamode metamaterial (the ‘reference’), (b) same, but with a rigid hollow cylinder (the ‘obstacle’) and (c) rigid hollow cylinder and cloaking shell (the ‘cloak’). For example, the homogeneous pentamode-metamaterial sample contains 16 × 8 × 8=1,024 face-centered cubic (fcc) extended unit cells with lattice constanta=125 μm and has a macroscopic total volume ofV=2 mm3, an important prerequisite for performing the measurements shown inFig. 3. Selected magnified views of the cloak in (c) are depicted in panels (d–f). Relevant dimensions are indicated (compareFig. 1b). Black scale bars, 200 μm. White scale bars, 10 μm. Figure 2: Fabricated elasto-mechanical structures. Electron micrographs of ( a ) the homogeneous pentamode metamaterial (the ‘reference’), ( b ) same, but with a rigid hollow cylinder (the ‘obstacle’) and ( c ) rigid hollow cylinder and cloaking shell (the ‘cloak’). For example, the homogeneous pentamode-metamaterial sample contains 16 × 8 × 8=1,024 face-centered cubic (fcc) extended unit cells with lattice constant a =125 μm and has a macroscopic total volume of V =2 mm 3 , an important prerequisite for performing the measurements shown in Fig. 3 . Selected magnified views of the cloak in ( c ) are depicted in panels ( d – f ). Relevant dimensions are indicated (compare Fig. 1b ). Black scale bars, 200 μm. White scale bars, 10 μm. Full size image In our quasi-static characterization experiments, a hard silicon stamp aligned parallel to the sample surface (see Fig. 3 ) pushes onto the sample via a motorized translational stage. The glass substrate at the bottom is fixed. We optically image the entire structure from the side, that is, in a plane perpendicular to the stamp, and record movies while varying the strain. To quantitatively analyse these movies, we use autocorrelation software to track individual points in the unit cells, delivering a spatial resolution beyond that of the individual camera pixels (for details see Methods). This analysis provides us with the displacement field or local-strain field directly from the experiment with good signal-to-noise ratio, even at maximum vertical strains (=vertical component of the displacement vector divided by the overall sample height) as low as 1%. 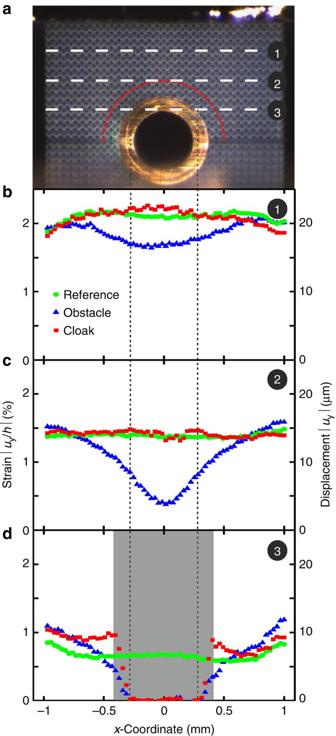Figure 3: Elasto-mechanical measurements. (a) Optical photograph (actually one movie frame) of the cloaking structure (seeFig. 2) when pushing is started from the top with a hard stamp. The red dashed semi-circle indicates the outer radius of the cloaking shell. The white dashed horizontal lines indicate the cuts depicted in panelsb(#1),c(#2) andd(#3). There, the vertical component of the displacement vectoruy(right-hand side scale) and the corresponding strain with respect to the overall sample heighth(left-hand side scale) are shown for the homogeneous pentamode metamaterial (‘reference’, green dots), the homogeneous pentamode metamaterial with a rigid hollow cylinder added (‘obstacle’, blue triangles) and for the cloak (red squares). With cloak (Fig. 1), we recover nearly a horizontal line, which we also find for a homogeneous medium without cylinder. This means that we have succeeded in making the hollow cylinder and its possible interior ‘unfeelable’. The region of the rigid cylinder (dashed lines) and the cloaking shell with near-zero displacement is highlighted in grey in panels (b–d). Figure 3: Elasto-mechanical measurements. ( a ) Optical photograph (actually one movie frame) of the cloaking structure (see Fig. 2 ) when pushing is started from the top with a hard stamp. The red dashed semi-circle indicates the outer radius of the cloaking shell. The white dashed horizontal lines indicate the cuts depicted in panels b (#1), c (#2) and d (#3). There, the vertical component of the displacement vector u y (right-hand side scale) and the corresponding strain with respect to the overall sample height h (left-hand side scale) are shown for the homogeneous pentamode metamaterial (‘reference’, green dots), the homogeneous pentamode metamaterial with a rigid hollow cylinder added (‘obstacle’, blue triangles) and for the cloak (red squares). With cloak ( Fig. 1 ), we recover nearly a horizontal line, which we also find for a homogeneous medium without cylinder. This means that we have succeeded in making the hollow cylinder and its possible interior ‘unfeelable’. The region of the rigid cylinder (dashed lines) and the cloaking shell with near-zero displacement is highlighted in grey in panels ( b – d ). Full size image Figure 3 shows the results for the homogeneous pentamode-metamaterial structure (the ‘reference’), the homogeneous pentamode structure with a rigid hollow cylinder (the ‘obstacle’) and the cloak including an additional pentamode-metamaterial shell. Data are shown for selected movie frames corresponding to the same strain of 2.8% at the top of the structures. Complete movies for the reference, the obstacle and the cloak are shown in Supplementary Movies 1, 2 and 3 , respectively. There (see Supplementary Fig. 2 ), we also show data for a different choice of d 2 / a =2.3% (instead of the above 2.4%) for a cloaking structure represented just like in Fig. 3 . These data provide information on the sensitivity of fabrication errors. Figure 3 displays the vertical strain along three selected horizontal lines. Most relevant is cut #2 located just slightly above the cloaking shell (indicated by the dashed semi-circle), where the displacement strongly varies for the obstacle structure: in the center, the modulus of the strain is nearly three times smaller than on the sides. This also means that one cannot simply cloak the obstacle by a homogeneous material, for example, by a block of some foam. In contrast, the displacement for the spatially inhomogeneous cloak structure is similar to that for a homogeneous environment without cylinder and without shell. Both displacement curves are just slightly bent towards the open sample sides. The other cut #1 further away from the rigid cylinder shows a similar behaviour, however, as to be expected, with much less pronounced differences between the homogeneous pentamode metamaterial and the obstacle in the first place, that is, there is less to be cloaked. This also means that the height of the structure is sufficiently large to avoid artifacts owing to finite sample height. Furthermore, from the fact that the above design process is based on an infinite depth of the cloak, whereas our fabricated structure is finite in depth as well, we estimate that artifacts due to measuring on the surface of the sample (actually about the first unit cell) rather than in the bulk are on the order of relative 10%. Likewise, the effects of the rigid cylinder are small for cut #3 as well. These overall observations mean that we have succeeded in approaching an ideal elasto-mechanical cloak. Comparison with numerical calculations Finally, we compare our experimental results with numerical continuum-mechanics calculations (for details see Methods) for the 3D pentamode microstructure to see how much possible experimental imperfections influence the results. Owing to memory and computation time constraints, we have not been able to perform calculations for the complete microstructure with 16 × 8 × 8 extended fcc unit cells. However, we have been able to obtain converged results for a reduced structure with 16 × 8 × 1 extended fcc unit cells and all of the above design parameters. In these calculations, we have employed fixed boundary conditions at the bottom substrate, have assumed zero horizontal component of the displacement vector at the top stamp and open-boundary conditions on the left and on the right—just like in the experiments discussed above and shown in Figs 2 and 3 . In the z -direction, we have used open-boundary conditions on one side (like in the experiment) and sliding-boundary conditions on the other. These mixed boundary conditions are an attempt to model the finite structure given tight numerical constraints. The numerical results in Fig. 4 are in good agreement with the experiments shown in Fig. 3 . In particular, the vertical component of the displacement vector just outside the cloaking shell in cut #2 already approaches a horizontal straight line—just like for a homogeneous pentamode-metamaterial environment. 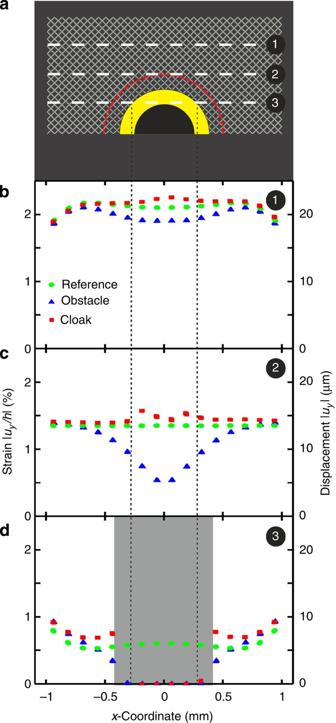Figure 4: Elasto-mechanical calculations. These theoretical results are represented like the experimental ones shown inFig. 3. The calculations use the pentamode microstructure identical to that depicted inFig. 1, but only 16 × 8 × 1 extended fcc unit cells. (a) Scheme, (b-d) cuts through the data along the three horizontal dashed straight lines indicated in panela. Figure 4: Elasto-mechanical calculations. These theoretical results are represented like the experimental ones shown in Fig. 3 . The calculations use the pentamode microstructure identical to that depicted in Fig. 1 , but only 16 × 8 × 1 extended fcc unit cells. ( a ) Scheme, ( b - d ) cuts through the data along the three horizontal dashed straight lines indicated in panel a . Full size image In 2006, Milton et al. [36] pointed out that the equations of solid elastostatics (and -dynamics) are not form-invariant under arbitrary curvilinear coordinate transformations. In sharp contrast, the Maxwell equations, the acoustic wave equation and the equations of heat conduction and diffusion are form-invariant. Their [36] mathematical finding suggests that perfect elastostatic cloaking may not be possible. Here, we have designed, fabricated and characterized an approximate elastostatic core-shell cloak based on 3D pentamode metamaterials. By using an autocorrelation-based image analysis to directly measure the displacement-vector field, we find very good cloaking performance under uniaxial pushing conditions. The fabrication of the underlying intricate cloaking microstructures with as many as 1,024 extended unit cells and with 2 mm 3 overall volume has only become possible by virtue of 3D dip-in galvo-scanner-based DLW optical laser lithography. Our results raise hopes that further mechanical metamaterial architectures may become accessible experimentally in the near future. Fabrication For the fabrication of the mechanical cloak as well as the reference structures, we used the commercially available DLW system Photonic Professional GT (Nanoscribe GmbH, Germany). In this setup, a liquid photoresist (IP-S resist, Nanoscribe GmbH) was polymerized via multi-photon absorption using a frequency-doubled Erbium fibre laser with a center wavelength of 780 nm and with a pulse duration of about 90 fs. The 3D exposure pattern was addressed by laser scanning using a set of galvo-mirrors and mechanical stages. The samples were prepared by drop-casting the negative-tone photoresist on a glass cover slip (22 × 22 × 0.17 mm). To avoid depth-dependent aberrations, the objective lens ( × 25, numerical aperture=0.8, Carl Zeiss) was directly dipped into the resist. Structural data were created in STL file format using the open-source software Blender and COMSOL Multiphysics. The software package Describe (Nanoscribe GmbH) was used to compile the CAD data into machine code. The scan raster was set to 0.5 μm laterally and 1 μm axially. The structure was laterally split into 8 scan fields of about 500 × 500 μm 2 footprint each that were stitched together. The writing speed was set to 5 cm s −1 . After the DLW of the preprogrammed pattern, the exposed sample was developed for 20 min in mr-Dev 600 and acetone. The process was finished in a supercritical point dryer to avoid capillary forces during drying. Sample characterization The images used for the extraction of the strain field were recorded with a camera (Sony GigE Vision XCG-5005CR) attached to a stereo microscope (Leica Mz 125 and a 0.5 × adapter from Leica mount to C-Mount). To reduce data, the images were then cropped to show only the structure and its close vicinity. For each picture taken, a linear stage induced a different predefined strain into the sample. The strain was successively increased in 50 steps towards the maximum value and afterwards decreased in 50 steps back to the initial value with a strain rate of 2% per minute. The glass substrate with the sample was attached to a goniometer and a micrometre stage to allow for positioning and aligning the sample with respect to the rest of the setup. The stamp was moved with a linear stage to which part of a silicon wafer with well-defined surface was attached. The software used to extract the strain field was based on a freely available package [37] . Here, selected markers with a set size of 15 × 15 image pixels were cross-correlated with the images from the measurement. The initial marker positions were fixed in a square grid with a spacing of 15 pixels in both dimensions spanning the entire size of the sample. This resulted in 67 markers along the horizontal direction and about 35 in the vertical. The tracking algorithm was set to a precision of 1/1,000 pixel. After cross-correlation, the position of each marker was known for each image. By subtracting the current marker positions from those of the reference frame, the displacement vector field was calculated for each image. Small movements of the glass substrate were corrected for. Movies of the reference, the obstacle and the cloak sample are given as Supplementary Movies 1–3 . There, the full displacement vectors, multiplied by a factor of 4, are depicted. Additional colour coding of the modulus of the displacement vector helps to identify gradients. Colour coding and scales are identical for the three movies. Numerical calculations We used the commercial software package COMSOL Multiphysics to numerically solve the static equations for linear elasticity. This means that neither a nonlinearity of the constituent material nor of the structure was accounted for. The geometry with the design parameters described in the main text was built using the internal kernel of COMSOL Multiphysics. The mesh consisted of about 640,000 tetrahedral elements (in COMSOL nomenclature: maximum element size=0.2 × a , minimum element size=0.05 × a , maximum element growth rate=16, resolution of curvature=0.7 and resolution of narrow regions=0.4) corresponding to 3–4 × 10 6 degrees of freedom. We used the direct solver MUMPS with a convergence tolerance of 10 −3 . As constituent material, we set an isotropic polymer with Young’s modulus=1 GPa , Poisson’s ratio v =0.4 and mass density ρ =1,200 kg m −3 . Owing to the scalability of the underlying equations, Young’s modulus and mass density did not even enter into the final results. The Poisson’s ratio was not actually important [28] , [29] . To deduce the displacements depicted in Fig. 4 , we have tracked the connections with diameter d in the middle of the extended fcc unit cell with respect to the z- direction. Further data processing was done like in the experiment. How to cite this article: Bückmann, T. et al. An elasto-mechanical unfeelability cloak made of pentamode metamaterials. Nat. Commun. 5:4130 doi: 10.1038/ncomms5130 (2014).